Hyperbolic spin vortices and textures in exciton–polariton condensates From cosmology to the microscopic scales of the quantum world, the study of topological excitations is essential for the understanding of phase conformation and phase transitions. Quantum fluids are convenient systems to investigate topological entities because well-established techniques are available for their preparation, control and measurement. Across a phase transition, a system dramatically changes its properties because of the spontaneous breaking of certain continuous symmetries, leading to generation of topological defects. In particular, attention is given to entities that involve both spin and phase topologies. Exciton–polariton condensates are quantum fluids combining coherence and spin properties that, thanks to their light-matter nature, bring the advantage of direct optical access to the condensate order parameter. Here we report on the spontaneous occurrence of hyperbolic spin vortices in polariton condensates, by directly imaging both their phase and spin structure, and observe the associated spatial polarization patterns, spin textures that arise in the condensate. Second-order phase transitions are accompanied by spontaneous symmetry breaking. A well-known example is the phase ordering occurring in atomic Bose–Einstein condensates [1] (BEC) and He 3 superfluids [2] . This abrupt and drastic change leads to the formation of topological defects, the properties and variety of which are determined by the nature of the order parameter and by broken continuous symmetries in the ordered phase. The Kibble–Zurek mechanism, first introduced in the context of cosmological theories [3] , was successfully transposed into the superfluid [4] , [5] and condensed matter domains [6] to account for the spontaneous formation of topological defects. This shows the high-degree of universality and interest of such studies. Particularly fascinating topological excitations are predicted to occur in spinor quantum fluids [7] and condensates [8] , where the additional spin degree of freedom allows for the existence of mixed spin-phase topologies. The possible occurrence of spin vortices and hedgehogs (magnetic monopole-like excitations) in spinor fluids has been predicted by several theorists [9] , [10] , [11] , [12] , [13] Such topological entities consist of quantized spin currents with no phase winding, when circumventing the vortex core. Recently, spontaneous chiral symmetry breaking, associated with occurrence of spin vortices, has been reported in a spinor BEC of 87 Rb atoms [14] . Up to now, proofs for the existence of magnetic monopole-like configurations have only been reported in spin-ice systems [15] , which would represent the counterpart of the fundamental Dirac magnetic monopoles, still elusive to observation as fundamental particles. These first studies paved the way to a new field of research, in the vast quantum fluids scientific community, devoted to the identification, characterization and understanding of spinor topologies. This is particularly true for polariton condensates [16] , [17] , where the vector order parameter can be accessed by optical means [18] . Interestingly, spin textures due to half-soliton formation have been recently observed in resonantly injected polariton fluids [16] and the motion of half-quantized vortices in an effective magnetic field has been predicted, suggesting an analogy with a magnetic charge [19] , [20] . In the broad field of semiconductor lasers and nonlinear optical media, spin vortices could be generated in engineered dedicated geometries, involving beam preparation or structure patterning [21] , [22] , [23] , [24] . Spontaneous appearance and stability of such vector vorticity has not been observed yet. Thus, the observation of spin vortices as spontaneous and stable entities still constitutes an experimental challenge, as it would also address theoretical predictions and the question about hedgehogs (monopoles) entropy instability. In this work, we assume and follow the original definition of ′t Hooft–Polyakov monopoles [25] , [26] or hedgehogs, as used by Volovik [7] in the theory of spinor condensates and chiral superconductors. Within such theoretical framework, we report experimental evidence of hyperbolic spin vortices, resulting from the spontaneous symmetry breaking associated to the onset of polariton condensation. The stabilization of the topological entities in the condensate steady state, achieved by the disorder in the BEC of polaritons, allows not only to identify different types of vortices but also to perform a complete study and unveil their specific properties. Spinor topological excitations Over the last few years, polariton quantum fluids have established themselves as a model system for the study of condensates [16] , [27] , [28] , [29] , superfluidity [30] and vorticity [18] , [31] , [32] . Polaritons arise as eigenmodes of the strong coupling regime between light and matter. This regime can be conveniently achieved in planar semiconductor microcavities, where the exciton resonance is efficiently coupled to the photon cavity mode [33] . Polaritons possess a pseudo-spin of ±1 (mapping to the σ + and σ − polarization of the emitted photon field), which allows for the spontaneous generation of spinor condensates—condensates with internal spin degree of freedom. A spinor condensate can be conveniently visualized as a BEC where two quasiparticle populations, with opposite spin, coexist and are mutually coherent. To reduce the strong repulsion of polaritons having the same spin (the polaritons with opposite spins are weakly interacting) the spinor polariton condensates are formed with equal populations of the spin-up and spin-down components, that is, with a linear polarization. The order parameter manifold of a spinor polariton condensate is M =( U (1) × S 1 )/ Z 2 and the order parameter can be written as a complex vector , where n ( r ) is the density of condensed polaritons. The total phase θ ( r ) is defined by the broken gauge U (1) symmetry, whereas the spontaneous polarization formation is given by the unit two-dimensional real vector d ( r ) (it defines the spin-quantization axis in the microcavity plane). The incomplete spin 1 basis in the case of polaritons results in the equivalence of the quantization axes of opposite directions (for example, x and − x ). The same ambivalence appears in the observable d , namely, the polarization of light. Nevertheless, this aspect does not prevent the experimental discrimination between the different kinds of spinor vortices. Moreover, in the case of polarization vortices, the phase of the condensate is constant and d ( r ) becomes the uniquely defined vector field. The intrinsic non-equilibrium nature of polariton condensates provides direct access to the condensate vector order parameter in a non-destructive way, through the measurement of the emitted photon field, which inherits the properties of the intracavity polariton field [34] . The isotropy group Z 2 reflects the fact that simultaneous transformations d →− d and θ → θ ±π leave the order parameter unchanged. This gives rise to possibility of formation of half-quantum vortices (HQVs) in polariton condensates, which involve rotations of both the phase and the polarization of the condensate at the same time. Expressing the condensate order parameter in the linear polarization basis, the HQV manifests as a π phase rotation and a π polarization rotation (half-integer rotations in units of 2π, hence their name). The two rotations combine together to ensure the global continuity of the wave function. An even more convenient way of visualizing a HQV is to consider the circular polarization basis. In this basis, the fractional vortical entity consists of an integer phase vortex appearing only in one spin component, whereas no vortex is found in the opposite spin component. A half vortex is therefore associated with a chiral symmetry breaking in the condensate. In polariton condensates, we understand the chiral symmetry as the symmetry between its left and right circular spin components and the related symmetry between the clockwise and counter-clockwise rotation of the linear polarization vector around a vortical entity. Thanks to advantageous properties of the polariton system, convincing experimental demonstration of HQVs has been reported [18] . More complex topological excitations—spin vortices and hedgehogs—are predicted to occur as superposition of HQVs in spinor polariton condensates [16] , making polariton condensates promising candidates for the study of spin topological entities and spin textures. The first homotopy group of the order parameter manifold is π 1 ( M )= Z × Z and the vortices in the polariton condensate are characterized by two winding numbers ( k , m ) for the polarization and phase rotations, respectively, expressed in units of 2π (a common notation, see for example, the study by Toledo-Solano et al. [16] ). These numbers can be either integer or half-integer simultaneously. It is convenient to think of HQVs as the fundamental building blocks of higher order vortex entities, namely, integer phase vortices and polarization vortices. In Fig. 1 , all the possible combinations of HQVs are schematically presented, indicating the sign of the phase winding for each spin component and the resulting integer topological entity. Phase vortices are identified by (0,±1), that is by a ±2π phase rotation when circumventing the vortex core. They correspond to the combination of and HQVs at the same spatial position. Polarization vortices (±1,0), instead, appear from the superposition of and HQVs. Such vortices are therefore characterized by a 2π rotation of the polarization and no phase rotation: the two spin components indeed feature counter-rotating phase windings (see Supplementary Fig. S2 ), which cancel out giving an overall flat phase for the condensate wave function. When considering integer excitations, while the phase vortices do not break the chiral symmetry of the system, as it is schematically shown in Fig. 1 , breaking of the chiral symmetry occurs in the case of the two allowed polarization vortices—hyperbolic spin vortices and hedgehogs. The sketch of the spin texture associated to each kind of polarization vortex unveils a fundamental difference between them. The hedgehog solution (+1,0) has a purely radial arrangement of polarization lines, characterized by C ∞ rotational symmetry, which resembles the magnetic field lines of a 't Hooft–Polyakov monopole [25] , [26] , [35] . Contrarily, the hyperbolic spin vortex (−1,0) gives rise to a mixed longitudinal-transverse field, with hyperbolic polarization lines, corresponding to a reduced C 2 discrete rotational symmetry, where two perpendicular main axes can be identified if a global change of phase by ±π is applied. 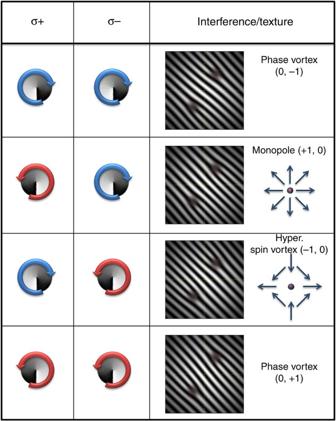Figure 1: Taxonomy of vortical entities. The table summarizes all the possible combinations of HQVs in the system. The arrows mimic the sense of rotation of the phase winding in each spin component. The resulting topological entities are classified in the last column, together with the expected interferometric signature from the PM interferometer (seeSupplementary Fig. S1). Note that the winding direction of a vortex maps to the orientation of the fork-like dislocation in the interferogram. For the polarization vortices, hedgehog (monopole) and hyperbolic spin vortices, a sketch of the polarization texture is given: the arrows represent the instant direction of the vector order parameter around the vortex core. Figure 1: Taxonomy of vortical entities. The table summarizes all the possible combinations of HQVs in the system. The arrows mimic the sense of rotation of the phase winding in each spin component. The resulting topological entities are classified in the last column, together with the expected interferometric signature from the PM interferometer (see Supplementary Fig. S1 ). Note that the winding direction of a vortex maps to the orientation of the fork-like dislocation in the interferogram. For the polarization vortices, hedgehog (monopole) and hyperbolic spin vortices, a sketch of the polarization texture is given: the arrows represent the instant direction of the vector order parameter around the vortex core. Full size image Here we report on the observation of hyperbolic spin vortices in a condensate of exciton–polaritons. We identify such entities using advanced interferometric techniques and performing a comprehensive experimental mapping of the real-space polarization structure of the condensate. The polarization-sensitive measurements allow us to get full access to the polarization texture imprinted in the condensate by the presence of the spin vortical entity. Our observations demonstrate the spontaneous breaking of the chiral symmetry for stable integer entities in a spinor polariton condensate. Vortex detection strategy As mentioned, a major advantage of polaritons is the direct access to the condensate vector order parameter through optical measurements. By using a polarization mixing (PM) interferometer (see Methods section) we are able to interfere with the σ + component of the condensate with a retroreflected replica of the orthogonal spin, the σ − component. Denoting as φ ±( x , y ) the σ + and σ − components of the order parameter, respectively, the retroreflection—centrosymmetric inversion–allows to overlap φ + ( x , y ) with φ − (− x ,− y ), where ( x , y )=(0,0) corresponds to the center of inversion. The use of such detection scheme has two major advantages that make it extremely convenient in the spinor condensate domain. On the one hand, the appearance of fringes in such an interferometric image is the signature of the mutual and long-range spatial coherence between the two spin components, proving the spinor nature of the condensate. On the other hand, the PM interferometer is sensitive to the sign of the phase windings of the spin components, mapping each type of topological excitation for our system to a unique and qualitatively different interferometric signature (see Fig. 1 ). This makes it possible to easily distinguish between phase vortices (0, ±1) and polarization vortices (±1, 0). Locating spin vortices The sample under examination is the same CdTe semiconductor microcavity used in our previous work [27] (see Methods section). We employ non-resonant optical excitation, ensuring that no coherence is imprinted to the polariton gas by the pump laser. We use an excitation density above the threshold for spontaneous BEC, exciting the system in a region of the sample where the polariton condensate is spinor in nature. In Fig. 2a and b the condensate density in σ + and σ − spin components, respectively, are shown. The large marker identifies the position of the vortex core, present in each spin. The interferogram, obtained by overlapping the two images, is shown in Fig. 2c . There, a clear pair of fork-like dislocations can be identified: the forks show the same orientation and are found at centrosymmetric positions with respect to the center of retroreflection. This is the expected interferometric signature of a spin vortex according to our detection scheme (see Supplementary Fig. S5 ). The corresponding phase structure, extracted via off-axis digital holographic techniques [36] (see Methods section), is shown in Fig. 2d : the position of the dislocations is even clearer and the direction of the phase windings is unveiled. The phase windings in the two spin components, around the vortex cores, are shown in Supplementary Fig. S2 . Further proof of the pure spin nature of the vortical entity is provided by analysis of the global condensate phase. This is done by interfering with the total condensate density image with an enlarged part of itself, acting as phase reference [37] . In the resulting interference pattern, the absence of fork-like dislocations at the position of the vortex shows that the global phase is indeed at rest (see Supplementary Fig. S3 ). The measured features nicely match those expected for a spin vortex entity of the two possible kinds (±1, 0). The sign of polarization rotation will be then assessed through the full characterization of the polarization structure of the topological defect, as discussed below. 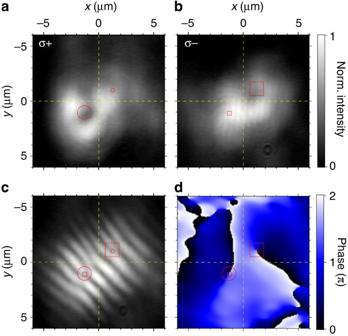Figure 2: Spin vortex interferometric signature. The real-space density ofσ+ (a) and the retroreflectedσ− (b) components of the condensate are overlapped in the PM interferometer to obtain the interference pattern (c). The corresponding phase structure is shown in (d). The polarization vortex interferometric signature consists in a pair of co-oriented fork-like dislocations, appearing at centrosymmetric positions with respect to the autocorrelation point. The red circle (forσ+) and square (forσ−) indicate the phase dislocation positions (large marker) and their corresponding centrosymmetric position (small marker). The yellow dashed lines cross at the autocorrelation point, central point of symmetry. Figure 2: Spin vortex interferometric signature. The real-space density of σ + ( a ) and the retroreflected σ − ( b ) components of the condensate are overlapped in the PM interferometer to obtain the interference pattern ( c ). The corresponding phase structure is shown in ( d ). The polarization vortex interferometric signature consists in a pair of co-oriented fork-like dislocations, appearing at centrosymmetric positions with respect to the autocorrelation point. The red circle (for σ +) and square (for σ −) indicate the phase dislocation positions (large marker) and their corresponding centrosymmetric position (small marker). The yellow dashed lines cross at the autocorrelation point, central point of symmetry. Full size image Assessing the spin textures A feature intrinsically associated to spin vortices is represented by their unique polarization texture. While phase vortices yield a zero net polarization rotation and no polarization pattern arises in the condensate, spin vortices consist in an integer (a 2π) rotation of the polarization when circumventing the vortex core. In order to extract the textures, we performed a full characterization of the polarization structure of the condensate at the spin vortex position (polariton density at the vortex core is shown in Fig. 3a ). We measure the Stokes parameters of the condensate emission along the horizontal–vertical (S 1 ), the diagonal (S 2 ) and the circular (S 3 ) bases (for a definition see Supplementary Note 1 ). The most striking and effective way of visualizing the presence of the integer spin rotation is to plot the linear polarization direction, calculated as tan −1 ( S 2 / S 1 ), around the spin vortex core. It is worth recalling that rotation angles in real space map by construction to a doubled rotation angle in the Stokes representation, so that the 2π winding of the spin vortex will result in a 4π rotation in the Stokes space. The result is plotted in Fig. 3b where indeed an anticlockwise rotation of the polarization around the core is clearly identified, matching in a really remarkable way the behavior expected from calculations ( Fig. 3c ). The slight distortion that appears in the spatial map, when going far from the vortex core, can be ascribed to the presence of disorder in the sample. As mentioned before, there are two possible kinds of polarization vortices: the monopole-like hedgehog (+1, 0) and the hyperbolic spin vortex (−1, 0). The anticlockwise rotation we found experimentally in the linear polarization angle allows solving the ambiguity between monopole (+1, 0) and spinning vortex (−1, 0) entity: it is the latter that matches with the observed texture. A hedgehog, with its radial polarization field would be associated with a clockwise rotation of the linear polarization angle instead (see sketch in Fig. 1 and Supplementary Fig. S6 ). 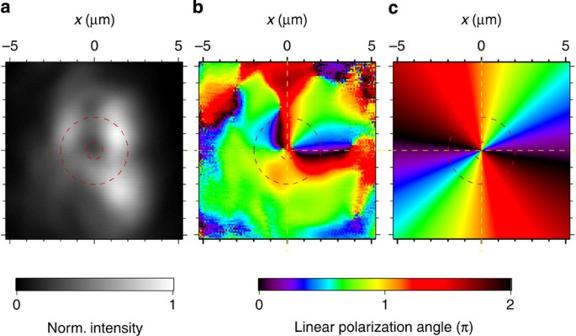Figure 3: Imaging of a spin vortex. (a) Time-integrated real-space condensate density. The core of the spin vortex can be identified at the center of the smaller red circle. (b) Linear polarization angle map, indicating the direction of the linear polarization, when circumventing the spin vortex core in the Stokes parameters space (by definition, a rotation of 2π in real space corresponds here to the doubled 4π rotation we observe). A good agreement is found between the experimental result and the theoretical simulation, which is shown in (c). The red dashed circles and the yellow lines serve as a guide for the eye to identify the vortex position. Figure 3: Imaging of a spin vortex. ( a ) Time-integrated real-space condensate density. The core of the spin vortex can be identified at the center of the smaller red circle. ( b ) Linear polarization angle map, indicating the direction of the linear polarization, when circumventing the spin vortex core in the Stokes parameters space (by definition, a rotation of 2π in real space corresponds here to the doubled 4π rotation we observe). A good agreement is found between the experimental result and the theoretical simulation, which is shown in ( c ). The red dashed circles and the yellow lines serve as a guide for the eye to identify the vortex position. Full size image The complete real-space characterization of the texture is presented in Fig. 4 . The polarization rates S 1 , S 2 and S 3 are shown in panels (a), (b) and (c), respectively. By comparing Fig. 4a and b one can notice that the extrema of S 1 correspond to zeros in S 2 and vice versa , as one would expect in the presence of a spin vortex. When analyzing the S 3 parameter, an intriguing and unexpected feature comes to the eye: a texture appears in the circular polarization basis as well ( Fig. 4c ). 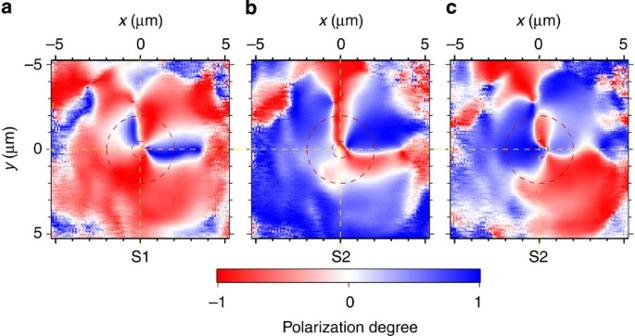Figure 4: Spin textures. Polarization rate (Stokes parameter) maps along the horizontal–vertical (a), diagonal (b) and circular (c) bases. The unpolarized emission has been removed (seeSupplementary Note 1andSupplementary Fig. S4). Figure 4: Spin textures. Polarization rate (Stokes parameter) maps along the horizontal–vertical ( a ), diagonal ( b ) and circular ( c ) bases. The unpolarized emission has been removed (see Supplementary Note 1 and Supplementary Fig. S4 ). Full size image An extremely convenient way of visualizing the measured polarization texture is by mapping the trajectory of the Stokes vector (S 1 , S 2 and S 3 ) in the Poincaré sphere when circumventing the spin vortex core. In such a representation, the ambivalence on the direction of the polariton spin quantization axis is suppressed due to the properties of the Stokes representation: the rotation of the Stokes vector is twice as the rotation of the real space quantization axis. Performing such a mapping one finds that indeed the Stokes vector undergoes a clear 4π rotation over a closed path, as shown in Fig. 5b . This rotation is not in the equatorial plane contrarily to the textbook theory of spin vortices. The actual trajectory is tilted with respect to an axis of the equatorial plane (red line in Fig. 5b ) towards the circular poles. 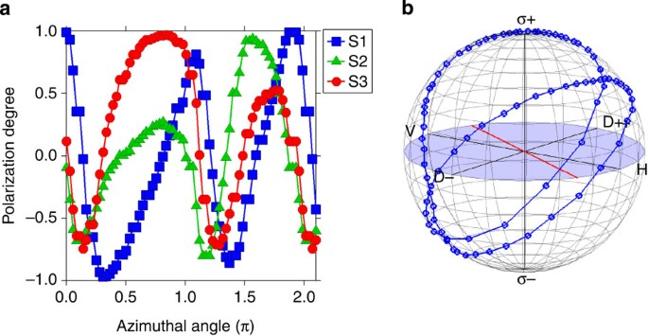Figure 5: Trajectories in the Poincaré sphere. (a) Polarization degree profiles around the vortex core the horizontal–vertical (S1), diagonal (S2) and circular (S3) bases. The unpolarized emission has been removed (seeSupplementary Fig. S4). (b) Representation in the Poincaré sphere of the double rotation of the Stokes vector of the condensate polarization, when circumventing the spin vortex core. Figure 5: Trajectories in the Poincaré sphere. ( a ) Polarization degree profiles around the vortex core the horizontal–vertical (S 1 ), diagonal (S 2 ) and circular (S 3 ) bases. The unpolarized emission has been removed (see Supplementary Fig. S4 ). ( b ) Representation in the Poincaré sphere of the double rotation of the Stokes vector of the condensate polarization, when circumventing the spin vortex core. Full size image The observed behaviour of the S 3 parameter is an unexpected feature for a spin vortex and comes from the influence a transverse-electric–transverse-magnetic (TE–TM) splitting of the polariton band. First, this splitting, together with the disorder potential of the microcavity, can lead to the appearance of a periodical S 3 variation at the edge of trapping potentials. This phenomenon is due to a radial flow of particles towards or from a point, similarly to the observation of spin Hall effect [38] . Second, TE–TM-splitting results in the metastability of the (−1, 0) vortex with respect to decay into a pair of and HQVs. As explained in the Supplementary Note 2 , these HQVs attract each other at short distances, when their cores overlap substantially, but they show a weak long-range repulsion due to the TE–TM splitting. As a result, the spin vortex decays into a pair of two separated HQVs, and , that are subject to the disorder potential present in the sample. The time-averaged motion of these half-vortices around each other in the presence of disorder leads to polarization maps shown in Fig. 4 . The formation of closely spaced pair of HQVs is reproduced by numerical simulations with a generalized Gross–Pitaevskii model [39] , [40] , where the exciton reservoir and the polariton condensation dynamics is taken into account (see Supplementary Note 3 ). In the simulations, assuming a shallow Gaussian potential trap, we observe the spontaneous appearance and pinning of spin vortices. In the case of polaritons, the interplay between gain–loss mechanism and disorder is the main responsible for the pinning and stabilization of the vortical entities, while the influence of a Kibble–Zurek like mechanism can be accounted for during their formation [41] , as previously introduced for ultracold atoms [5] , still the object of interest in recent experiments [42] . In the polariton context, we refer to such Kibble–Zurek like mechanism from a phenomenological point of view, in relation to the behavior of condensate formation as from theoretical simulations. Out of initial noise conditions, random nucleation islands form at the early instants of the condensate formation. The initially small, disconnected regions then expand in space and merge together, locking in phase and becoming mutually coherent with each other. Out of their merging, quantized vorticity is seen to form in the system. If birefringence is introduced in the calculation (which is a common feature associated to disorder in the sample), the discrete symmetry of the hyperbolic spin vortices leads to the pinning of the spin texture along the birefringence axes. Moreover, the HQVs in the two opposite spin components, forming the spin vortex, do not get pinned exactly at the same position inside the trap even within calculation times of 10 ns. This separation results in quite strong spin texture in S 3 , while S 1 and S 2 spin textures are not much affected. This particular feature is extremely dependent on the pinning dynamics, that is to say, on the disorder landscape. We found that the calculated S 1 , S 2 and S 3 parameters ( Supplementary Figs S7 and S8 ) qualitatively match the relevant features of the experimental ones of Fig. 4 . In this work we have proved the existence of rare spinor vortical entities, the so-called hyperbolic spin vortices, spontaneously arising in non-equilibrium polariton condensates with spin degree of freedom. The direct measurement of the characteristic spin texture, associated to the topological defect, strengthens and completes the observation. This observation highlights once more the pertinence and growing interest of polariton condensates, within the quantum fluids community, as complex and rare topological defects can be completely characterized by optical means thanks to the unique features of such quasiparticles. Furthermore, the optical access to the condensate order parameter makes it also possible to envisage deterministic control and manipulation of the spin vortical entities by external laser fields. The very mechanism of chiral symmetry breaking underlying the formation of the hyperbolic spin vortices is also at the basis of the so far untraceable monopole-like hedgehog. Further investigations are required to identify experimental conditions that would stabilize these rare entities in a polariton quantum fluid, possibly through engineering of appropriate potential traps in microcavity samples. Future experiments may also concentrate on the dynamics of formation of spinor vortices, conceivably unveiling further insights on the chiral symmetry breaking we observe. Sample The sample is a CdTe planar semiconductor microcavity containing 16 quantum wells and featuring 26 meV of Rabi splitting, which was used in our previous work [27] . As a result of the growth process, the sample features a disorder potential that is is felt by polaritons. In some regions of the sample, such disorder landscape is responsible for the pinning of vortical entities within the condensate, both fractional (HQVs) [18] and integer phase vortices. In this work we present the even more exotic and intriguing spin vortical entities, pinned in the two-component polariton condensate. Phase-extraction technique Using digital holographic techniques, starting from the interference pattern in real space, it is possible to extract the phase structure of the condensate. Schematically: the interferogram image is transformed with a two-dimensional (2D) FFT algorithm into a reciprocal space map. Because of the applied interference fringes, the oscillatory part carrying the phase information can be isolated in reciprocal space in order to extract the phase information. Eventually, to obtain the polariton condensate phase, a reference phase corresponding to the fringe pattern imposed by the interferometer geometry is subtracted. Polarization mixing interferometer A schematic depiction of the experimental setup, consisting in a photoluminescence (PL) detection scheme in reflection configuration, is shown in Supplementary Fig. S1 . We excite the system using a non-resonant Ti:Sapphire quasi-CW laser, detuned to ~45 nm above the polariton resonance, which is focused down onto the surface of the sample through a 0.5 NA microscope objective. The same objective collects the condensate emission that is sent through a λ /4 wave plate, which transforms the circular polarization components of the PL signal into cross-linear ones. The signal is then used as input in our PM interferometer. In this interferometer, a polarizing beam splitter separates the two linear polarization components. In one of the arms, the signal is left untouched (the one corresponding to the σ + component). On the contrary, in the other arm (corresponding to the σ −) the polarization is rotated by 90° using a λ /2 wave plate, to make it collinear with the one of the σ + arm. The σ − component is then retroreflected, realizing a centrosymmetric replica of it. The signal of the two arms is then overlapped at the output of the interferometer and imaged in real-space on a CCD camera. Overall, the PM interferometer realizes the interference of the σ + component of the condensate with a centrosymmetric replica of the σ − one. The appearance of fringes at the output of the PM interferometer is the signature of the mutual coherence between the two spin components of the condensate, confirming the spinor nature of the condensate. A fundamental advantage of the PM interferometer is the univocal mapping of each allowed topological excitation to a specific and qualitatively different interferometric signature (as shown in Fig. 1 : interference patterns in the third column). It should be noted that for a given and known interference position, the signature of the two spin vortex solutions is in principle distinguishable. Nevertheless, it should be noted that the orientation of the fork-like dislocations in the interferogram depends also on the interference wavevector, which is imposed by the geometry of the interferometer. Of course, it holds that for any fixed orientation of the interference fringes, the two vortical entities of spin will have opposite fork orientations and therefore a different signature, but from the practical point of view one does not have any reference to discriminate between the two configurations. In fact, the complexity of the experimental set-up prevents us from having a straightforward reference frame to label the directions of the fork-like dislocations. It is therefore more rigorous and reliable to extract such information from the full characterization of the polarization textures through polarization-resolved measurements. The identification then consists in identifying the direction of rotation of the linear polarization around the vortex core in a fixed (H,V,D+,D−, σ +, σ −) measurement frame. Polarization-resolved measurement To experimentally determine the spin texture we performed real-space measurements of the condensate density with polarization resolution. The PL signal—the condensate density ( Fig. 4a )—is analysed along the horizontal, vertical, diagonal and anti-diagonal linear polarization direction, by sending it through a λ /2 wave plate and a linear polarizer (Glan prism) just before imaging on the CCD camera. This allows determining S 1 and S 2 parameters. By use of a λ /4 wave plate the circular polarization rate S 3 is also measured. By choosing the orientation of the linear polarizer, we are able to perform accurate polarization-resolved condensate density measurements. This allows reconstructing the polarization pattern—texture—around the spin vortex core. The complete characterization of the polarization map of the condensate allows to discriminate between the occurrence of a hedgehog vortex (+1, 0) and a hyperbolic spin vortex (−1, 0), by analysis of the sense of rotation of the vortex trajectory in the Poincaré sphere, as discussed in the main body of the paper. How to cite this article: Manni, F. et al. Hyperbolic Spin Vortices and Textures in Exciton-Polariton Condensates. Nat. Commun. 4:2590 doi: 10.1038/ncomms3590 (2013).